Expansion–contraction of photoresponsive artificial muscle regulated by host–guest interactions The development of stimulus-responsive polymeric materials is of great importance, especially for the development of remotely manipulated materials not in direct contact with an actuator. Here we design a photoresponsive supramolecular actuator by integrating host–guest interactions and photoswitching ability in a hydrogel. A photoresponsive supramolecular hydrogel with α-cyclodextrin as a host molecule and an azobenzene derivative as a photoresponsive guest molecule exhibits reversible macroscopic deformations in both size and shape when irradiated by ultraviolet light at 365 nm or visible light at 430 nm. The deformation of the supramolecular hydrogel depends on the incident direction. The selectivity of the incident direction allows plate-shaped hydrogels to bend in water. Irradiating with visible light immediately restores the deformed hydrogel. A light-driven supramolecular actuator with α-cyclodextrin and azobenzene stems from the formation and dissociation of an inclusion complex by ultraviolet or visible light irradiation. The construction of actuators, which are reminiscent of artificial muscles, is an important target in fields ranging from medicine to physics, materials science and materials engineering. One research topic to realize muscle-like movements in actuators is converting input energies (electric, thermal, charge, photo energies) into visualized movements (deformation, transformation, pressure, and so on) [1] , [2] , [3] . Many attempts have been made to realize organic, inorganic, electrostrictive and piezoelectric materials [4] , [5] , [6] , [7] . Polymer-based actuators (polymer gel [8] , [9] , [10] , [11] , liquid crystalline elastomers [12] , [13] , [14] , [15] , [16] , [17] , [18] , [19] , [20] , [21] , [22] , [23] , conjugated polymers [24] and carbon nanotubes [25] , [26] , [27] , [28] ) show reversible shape deformations in response to external stimuli. However, there are no examples of ‘artificial muscles’ in which polymeric materials are able to expand and contract owing to stimulus-responsive host–guest interactions. If such systems are realized, they can be used not only to confirm the mechanism for biological movement but also to realize ‘soft robotics’. Previously, we have reported that stimulus-responsive supramolecular polymers are formed by mixing an aqueous solution of a host polymer containing cyclodextrin (CD) with that of a guest polymer containing azobenzene (Azo) [29] , [30] , [31] , [32] or ferrocene [33] . An external stimulus induces a sol–gel phase transition in these hydrogels. Formation of inclusion complexes acts as crosslink points for the polymers to yield supramolecular hydrogels, whereas decomposition of inclusion complexes yields the sol state. We hypothesized that if covalent bonds partly crosslink polymer chains, then external stimuli would induce an expansion–contraction behaviour, and not a sol–gel phase transition. However, to our knowledge, there are no reports on an external stimulus-responsive host–guest gel with expansion–contraction properties. Theoretically, the ionic strength and crosslink densities (effective network chain) have important roles in the expansion–contraction ability of hydrogels [34] , [35] . Although previous papers have altered the expansion–contraction properties of hydrogels via ionic strengths, changing these properties using the crosslink density in a host–guest complex has yet to be reported. We selected Azo compounds as guest molecules because the association constant of α-cyclodextrin (αCD) for trans -azobenzene ( trans -Azo) is larger than that for cis -azobenzene ( cis -Azo) ( trans -Azo; K a =12,000 M −1 , cis -Azo; K a =4.1 M −1 ) [30] , [31] ; Azo affects the photoinduced deformation and remote controllability. Herein, we report supramolecular materials with expansion and contraction abilities constructed by host–guest polymers. Using supramolecular hydrogels, which exhibit an expansion–contraction behaviour that depends on the photostimulus, we successfully prepared a photostimulus-responsive supramolecular actuator reminiscent of a natural muscle. Preparation of an expansion–contraction gel Initially we prepared a host–guest gel (αCD–Azo gel) with αCD and Azo ( Supplementary Methods ). αCD–Azo gel is synthesized by radical copolymerization of a mixture of αCD-modified acrylamide (αCD–AAm), azobenzene acrylamide (Azo–AAm), methylene bisacrylamide (MBAAm) and acrylamide (AAm) in dimethyl sulphoxide (DMSO). The mole percentage contents ( x ) of αCD–AAm and Azo–AAm units are x =1–3 mol%. The polymer chains in αCD–Azo gel are crosslinked with MBAAm (the mole percentage content of MBAAm: y =2 and 4 mol%). 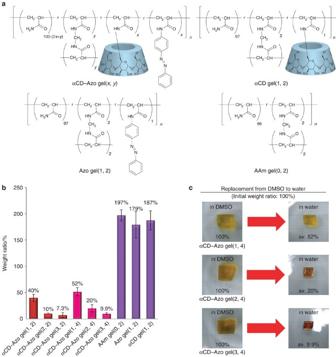Figure 1: Polymer gels used to prepare photoresponsive supramolecular actuators and their expansion–contraction behaviour. (a) Chemical structures of αCD–Azo gel, αCD gel (without the Azo–AAm unit), Azo gel (without the αCD–AAm unit) and AAm gel (without αCD–AAm and Azo–AAm units).xis the mole percentage of the host and guest units.yis the mole percentage of the crosslinking unit (MBAAm). (b) Weight ratio change in the gels upon replacing DMSO with water. Gels initially absorb DMSO. The weight ratio of gel absorbed with DMSO is defined as 100%. Error bars, standard deviation for 5 measurements. (c) Photographs of the volume change of αCD–Azo gel (x, 4) upon replacing DMSO with water. Av., average. Figure 1a depicts the chemical structures of αCD–Azo gel( x , y ), αCD gel(1, 2) (without the Azo–AAm unit), Azo gel(1, 2) (without the αCD–AAm unit) and AAm gel(0, 2) (without αCD–AAm and Azo–AAm units). 1 H solid state NMR ( 1 H magic angle spinning NMR ( 1 H MAS-NMR)) and infrared spectroscopy characterized the chemical structure of αCD–Azo gels ( Supplementary Figs S1 and S4 ), Azo gel(1, 2) ( Supplementary Figs S2 and S4 ) and AAm gel(0, 2) ( Supplementary Figs S3 and S4 ). Figure 1: Polymer gels used to prepare photoresponsive supramolecular actuators and their expansion–contraction behaviour. ( a ) Chemical structures of αCD–Azo gel, αCD gel (without the Azo–AAm unit), Azo gel (without the αCD–AAm unit) and AAm gel (without αCD–AAm and Azo–AAm units). x is the mole percentage of the host and guest units. y is the mole percentage of the crosslinking unit (MBAAm). ( b ) Weight ratio change in the gels upon replacing DMSO with water. Gels initially absorb DMSO. The weight ratio of gel absorbed with DMSO is defined as 100%. Error bars, standard deviation for 5 measurements. ( c ) Photographs of the volume change of αCD–Azo gel ( x , 4) upon replacing DMSO with water. Av., average. Full size image αCD–Azo gels feature three types of gels with host–guest units ( x =1, 2 and 3 mol%) and crosslinking units ( y =2 and 4 mol%). After gelation in DMSO, rinsing with water replaces the absorbed DMSO in the αCD–Azo gel( x , y ). Figure 1b depicts the weight ratio of the gels upon substituting DMSO with water. The weight ratio of gel absorbed with DMSO is defined as 100%. Removing the absorbed DMSO significantly decreases the weight ratio of αCD–Azo gel( x , y ) with an increase in the mol% of the αCD and Azo unit. As shown in Fig. 1c , substituting DMSO with water causes αCD–Azo gel( x , 4) to contract. In addition, the weights of αCD–Azo gel(2, 2) and (3, 2) decrease, reaching 10±1.1 and 7.3±4.7% of the initial weight, respectively. αCD–Azo gel( x , 2 ) with 2 mol% of MBAAm exhibits a greater contraction than αCD–Azo gel( x , 4) with 4 mol% of MBAAm. On the other hand, the weight ratio of αCD gel(1, 2), Azo gel(1, 2) and AAm gel(0, 2) increase upon solvent manipulation, reaching 197±11, 179±25 and 187±18% of their original weights, respectively ( Fig. 1b ). αCD–Azo gel( x , y ) contracts upon substituting DMSO with water because host–guest complexation forms crosslinks, which was confirmed using creep rupture measurements. Supplementary Figure S5 shows the stress–strain curves of αCD–Azo gel( x , 2) with various amounts of host–guest units. The stress of αCD–Azo gel( x , 2) increases as αCD and the Azo units ( x ) increase. These results indicate that the formation of an inclusion complex between αCD and the Azo units causes αCD–Azo gels to shrink owing to the increase in crosslinks. Expansion of αCD–Azo gel with competitive molecules To demonstrate the complementary host–guest interaction between αCD and the Azo groups, αCD–Azo gels were immersed in aqueous solutions of competitive guest or host molecules for 12 h. We chose diol derivatives as competitive guest molecules (for example, 1,4-butane diol (C 4 diol), 1,5-pentane diol (C 5 diol), 1,6-hexane diol (C 6 diol) and 1,7-heptane diol (C 7 diol)) [36] . Flat plates of αCD–Azo gels (size: 3 × 3 × 2 mm 3 ) were immersed in solutions with various concentrations of competitive guests or hosts. 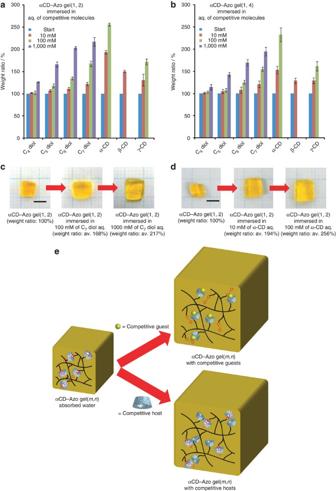Figure 2: Expansion of αCD–Azo gels immersed in aqueous solutions of competitive molecules. (a) Weight ratio change of the αCD–Azo gel(1, 2) immersed in aqueous solutions of competitive molecules such as 1,4-butane diol (C4diol), 1,5-pentane diol (C5diol), 1,6-hexane diol (C6diol), 1,7-heptane diol (C7diol) and competitive hosts (CDs). Concentration of competitive molecules in water was changed from 0 to 1,000 mM. Data for 1,000 mM of αCD and γCD are not collected because they become saturated at 100 mM. Saturated concentration of βCD is 10 mM. Error bars, standard deviation for 5 measurements. (b) Weight ratio change of αCD–Azo gel(1, 4) immersed in competitive molecules. Error bars, standard deviation for 5 measurements. (c) Photographs of the volume change of αCD–Azo gel(1, 2) immersed in aqueous solutions of C7diol. Scale bar, 5mm. (d) Photographs of the volume change of αCD–Azo gel(1, 2) immersed in aqueous solutions of αCD. Scale bar, 5mm. (e) Schematic illustration of the expansion of αCD–Azo gels immersed in aqueous solutions of competitive molecules. Azo unit on the polymer chain is ejected from the αCD cavity by competitive guests. Added CDs competitively form inclusion complexes with the Azo units. Av., average. Figure 2a and b show the weight ratio of αCD–Azo gel(1, 2) or αCD–Azo gel(1, 4) with competitive guests or competitive hosts. In addition, we investigated the influence of the concentration of competitive molecules on the weight ratio of αCD–Azo gels. After immersion in an aqueous solution of competitive guests for 12 h, the weight ratio of the αCD–Azo gels depends on the association constant with αCD [36] as well as the concentration of competitive guests. When αCD–Azo gels(1, 2) are immersed in 100 and 1,000 mM of C 7 diol aq., the weight ratio of αCD–Azo gel(1, 2) after 12 h are 168±6.0 and 217±9.5% of the original weight ratio, respectively ( Fig. 2c ). The weight ratio of αCD–Azo gel(1, 2) is larger than that of αCD–Azo gel(1, 4), indicating that the smaller the crosslink ratio of αCD–Azo gels leads to the greater the change in volume. Immersing αCD–Azo gels(1, 2) in 10 and 100 mM of αCD aq. leads to a 194±4.2 and 256±3.5% increase in the weight ratio, respectively ( Fig. 2d ). The weight ratio of αCD–Azo gel(1, 2) immersed in αCD aq. is larger than those of βCD and γCD aq. owing to the low affinities of βCD and γCD for Azo derivatives [36] . The expansion of αCD–Azo gels depends on the association constant of the competitive molecules with host or guest units on the polymer chains. These results indicate that αCD–Azo gels shrink in water owing to the formation of an inclusion complex between αCD and the Azo units, and then competitive molecules decompose the inclusion complexes, which function as crosslinkers, to swell αCD–Azo gels ( Fig. 2e ). Figure 2: Expansion of αCD–Azo gels immersed in aqueous solutions of competitive molecules. ( a ) Weight ratio change of the αCD–Azo gel(1, 2) immersed in aqueous solutions of competitive molecules such as 1,4-butane diol (C 4 diol), 1,5-pentane diol (C 5 diol), 1,6-hexane diol (C 6 diol), 1,7-heptane diol (C 7 diol) and competitive hosts (CDs). Concentration of competitive molecules in water was changed from 0 to 1,000 mM. Data for 1,000 mM of αCD and γCD are not collected because they become saturated at 100 mM. Saturated concentration of βCD is 10 mM. Error bars, standard deviation for 5 measurements. ( b ) Weight ratio change of αCD–Azo gel(1, 4) immersed in competitive molecules. Error bars, standard deviation for 5 measurements. ( c ) Photographs of the volume change of αCD–Azo gel(1, 2) immersed in aqueous solutions of C 7 diol. Scale bar, 5mm. ( d ) Photographs of the volume change of αCD–Azo gel(1, 2) immersed in aqueous solutions of αCD. Scale bar, 5mm. ( e ) Schematic illustration of the expansion of αCD–Azo gels immersed in aqueous solutions of competitive molecules. Azo unit on the polymer chain is ejected from the αCD cavity by competitive guests. Added CDs competitively form inclusion complexes with the Azo units. Av., average. Full size image Photoresponsive volume change of αCD–Azo gels We investigated the effects of photostimuli on the expansion–contraction behaviour of αCD–Azo gels by irradiating flat plates of αCD–Azo gels (size: 5–6 × 5–6 × 2–3 mm 3 ) immersed in water for an hour. Photoirradiation with ultraviolet light ( λ =365 nm) isomerizes the trans -Azo group into the cis -Azo group, whereas the reverse occurs with visible (Vis) light ( λ =430 nm) [37] . 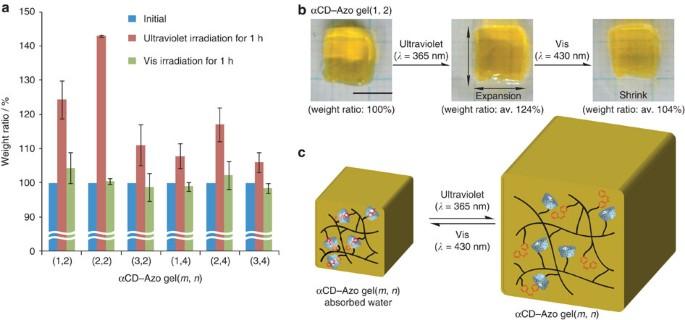Figure 3: Photoresponsive weight change of αCD–Azo gels in water. (a) Weight change of αCD–Azo gels before and after photoirradiation with ultraviolet light (λ=365 nm) and Vis light (λ=430 nm). Error bars, standard deviation for 5 measurements. (b) Photographs of the volume change of αCD–Azo gel(1, 2) irradiated by ultraviolet and Vis light. Scale bar, 5 mm. (c) Schematic illustration of the expansion–contraction of αCD–Azo gel irradiated by ultraviolet and Vis light. After ultraviolet irradiation, which induces isomerization from thetrans- tocis-form, the complex between αCD and Azo units decomposes to expand αCD–Azo gels. Vis irradiation causes isomerization from thecis- totrans-form, and complexation between αCD and the Azo units regenerates, shrinking the αCD–Azo gel. Av., average. Figure 3a shows the weight change of αCD–Azo gels upon ultraviolet and Vis light irradiation. The light source located above the gels had a 300W Xenon lamp with a mirror module and band-pass filters to irradiate at a suitable wavelength. Ultraviolet irradiation of αCD–Azo gels increases the weight of the hydrogels, whereas continuous irradiation of Vis light to the αCD–Azo gels restores the initial weight and volume. These volume changes of αCD–Azo gels are correlated with the inclusion complex formation between αCD and Azo units ( Fig. 3b ). The association constant of αCD for trans -Azo is larger than that for cis -Azo [30] , [31] . The difference in the association constants of αCD for the Azo isomers creates the expansion–contraction behaviour in αCD–Azo gels upon ultraviolet and Vis light irradiation. Figure 3: Photoresponsive weight change of αCD–Azo gels in water. ( a ) Weight change of αCD–Azo gels before and after photoirradiation with ultraviolet light ( λ =365 nm) and Vis light ( λ =430 nm). Error bars, standard deviation for 5 measurements. ( b ) Photographs of the volume change of αCD–Azo gel(1, 2) irradiated by ultraviolet and Vis light. Scale bar, 5 mm. ( c ) Schematic illustration of the expansion–contraction of αCD–Azo gel irradiated by ultraviolet and Vis light. After ultraviolet irradiation, which induces isomerization from the trans - to cis -form, the complex between αCD and Azo units decomposes to expand αCD–Azo gels. Vis irradiation causes isomerization from the cis - to trans -form, and complexation between αCD and the Azo units regenerates, shrinking the αCD–Azo gel. Av., average. Full size image The weight ratio of αCD–Azo gel( x , 2) with 2 mol% of MBAAm is larger than that of αCD–Azo gel( x , 4) with 4 mol% of MBAAm, indicating that a smaller crosslinking ratio induces a larger volume change in the gel. Similarly, the weight ratio of αCD–Azo gel(2, 2) is larger than that of αCD–Azo gel(3, 2). The inside of the Azo unit of αCD–Azo gel(3, 2) does not isomerize from the trans - to cis -form because the concentration of the Azo group is too high to optically transmit through the opposite side, meaning ultraviolet light is absorbed on the surface of αCD–Azo gel(3, 2). On the other hand, the weight ratio of βCD–Azo gel(1, 2) does not change with the irradiation because the association constants of βCD with trans -Azo and cis -Azo are comparable. These results indicate that the change in the photoresponsive volume of αCD–Azo gels is due to the extensive complementarity between the αCD and trans -Azo units. We used ultraviolet–Vis spectroscopy ( Supplementary Figs S6 and S7 ) to track the photoisomerization of the Azo group. As the irradiation time at λ =365 nm increases, the intensity of π–π* transition band of the Azo group in αCD–Azo gel(1, 2) decreases and an n –π* transition band appears. Conversely, as the Vis irradiation time at λ =430 nm increases, cis -Azo recovers the intensity of π–π* transition band around 350 nm and the n–π* transition band disappears. These results indicate that ultraviolet irradiation causes the trans -Azo group of the αCD–Azo gel to isomerize into the cis -form, whereas Vis irradiation causes the cis -Azo group to isomerize into the trans -form. We characterized the trans - and cis -contents of the αCD–Azo gels by calculating the integral value of the Azo unit with 1 H MAS-NMR ( Supplementary Fig. S8 ). Before ultraviolet irradiation, the isomer contents of αCD–Azo gel is trans : cis =70±2.2:30±2.2, whereas afterward, the ratio changes to trans:cis =5±1.2:95±1.2. However, the isomer contents recovers to trans : cis =69±0.57:31±0.57 upon Vis light irradiation ( Supplementary Fig. S8 ). Consequently, the photoisomerization of the Azo unit is reversible even in the αCD–Azo gel. Figure 3c shows the proposed scheme for the expansion–contraction behaviour of αCD–Azo gels by photoirradiation. Before photoirradiation, αCD–Azo gels contract forcefully to form supramolecular noncovalent crosslinks between αCD and trans -Azo units through host–guest interactions. After ultraviolet irradiation ( λ =365 nm), the trans -form isomerizes into the cis -form, decreasing the number of noncovalent crosslinks as the inclusion complexes between αCD and the Azo units decompose, causing the αCD–Azo gels to expand. However, after subsequent Vis irradiation ( λ =430 nm) the trans -form recovers, increasing the number of noncovalent crosslinks and forming inclusion complexes, which causes αCD–Azo gels to contract. Thus, the expansion–contraction process of these supramolecular hydrogels depends on the wavelength. Photoresponsive actuator of αCD–Azo gels We prepared photoresponsive actuators using the expansion–contraction ability of αCD–Azo gels. 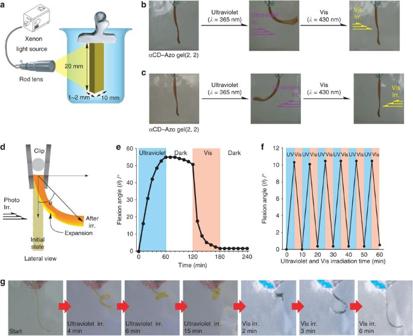Figure 4: Photoresponsive actuator of αCD–Azo gel in water. (a) Experimental devices and the size of αCD–Azo gel(2, 2) in water. (b) Light irradiation from the left side of αCD–Azo gel(2, 2) for an hour. After ultraviolet irradiation, αCD–Azo gel(2, 2) bends to the right side. Subsequent irradiation with Vis light restores the initial state. (c) Light irradiation from the right side of αCD–Azo gel(2, 2) for an hour. After ultraviolet irradiation, αCD–Azo gel(2, 2) bends to the left side. Subsequent irradiation with Vis light restores the initial state. (d) Lateral view of αCD–Azo gel(2, 2) hung with a clip. Flexion angle (θ) is defined here. (e) Plots of irradiation time versus the flexion angle (θ) in αCD–Azo gel(2, 2). Blue and red areas denote ultraviolet irradiation and Vis irradiation, respectively. Blank area indicates dark storage without light irradiation. Flexion angle (θ) is measured using snapshots. (f) The repeated experiment of αCD–Azo gel(2, 2) irradiated with ultraviolet and Vis lights for 5 min. Plots show the correlation between irradiation time and flexion angle (θ). (g) Light irradiation from the left side of the ribbon-shaped αCD–Azo gel(1, 2) for 15 min. After ultraviolet irradiation, αCD–Azo gel(1, 2) forms a coil. Subsequent irradiation with Vis light restores the initial state. The colour profile of pictures under Vis light irradiation is adjusted to create clear images. The actual movie is shown inSupplementary Movie 8. Figure 4a shows a component drawing of an αCD–Azo gel actuator where the plate gel is 20 × 10 × 1–2 mm 3 . We chose αCD–Azo gel(2, 2). Irradiating the plate gel with ultraviolet light ( λ =365 nm) from the left side bends the gel to the right, whereas irradiating the bent gel with Vis light ( λ =430 nm) from the same side for an hour restores the initial condition ( Fig. 4b ). Similarly, irradiating the plate gel from the right side causes the gel to bend to the left side, while irradiating with Vis light restores the initial state ( Fig. 4c ). This bending behaviour can be repeated for at least five cycles with varying strains. These results demonstrate that αCD–Azo gels bend in the opposite direction of the incident light. Figure 4: Photoresponsive actuator of αCD–Azo gel in water. ( a ) Experimental devices and the size of αCD–Azo gel(2, 2) in water. ( b ) Light irradiation from the left side of αCD–Azo gel(2, 2) for an hour. After ultraviolet irradiation, αCD–Azo gel(2, 2) bends to the right side. Subsequent irradiation with Vis light restores the initial state. ( c ) Light irradiation from the right side of αCD–Azo gel(2, 2) for an hour. After ultraviolet irradiation, αCD–Azo gel(2, 2) bends to the left side. Subsequent irradiation with Vis light restores the initial state. ( d ) Lateral view of αCD–Azo gel(2, 2) hung with a clip. Flexion angle ( θ ) is defined here. ( e ) Plots of irradiation time versus the flexion angle ( θ ) in αCD–Azo gel(2, 2). Blue and red areas denote ultraviolet irradiation and Vis irradiation, respectively. Blank area indicates dark storage without light irradiation. Flexion angle ( θ ) is measured using snapshots. ( f ) The repeated experiment of αCD–Azo gel(2, 2) irradiated with ultraviolet and Vis lights for 5 min. Plots show the correlation between irradiation time and flexion angle ( θ ). ( g ) Light irradiation from the left side of the ribbon-shaped αCD–Azo gel(1, 2) for 15 min. After ultraviolet irradiation, αCD–Azo gel(1, 2) forms a coil. Subsequent irradiation with Vis light restores the initial state. The colour profile of pictures under Vis light irradiation is adjusted to create clear images. The actual movie is shown in Supplementary Movie 8. Full size image In addition, we investigated the influence of irradiation time (1, 5, 10, 20, 30 and 60 min.) on the amount of the flexion angle in αCD–Azo gel(2, 2) ( Fig. 4e and Supplementary Figs S9 and S10 ). Figure 4d defines the flexion angle ( θ ), and Supplementary Movies 1 , 2 , 3 , 4 , 5 , 6 depict the flex behaviour of αCD–Azo gel(2, 2). Figure 4e shows the flexion angle of αCD–Azo gel(2, 2) irradiated with ultraviolet and Vis lights for an hour. The flexion angle ( θ ) becomes saturated after ultraviolet irradiation for about an hour, and does not significantly decrease upon standing under its own weight for an hour in the dark. Conversely, irradiation with Vis light for an hour restores the bent gel to the initial state and the flexion angle decreases. The Vis irradiation time required for the bent gel to return to a flat gel is similar to the ultraviolet irradiation time. Figure 4f and Supplementary Movie 7 show the repeated experiment of αCD–Azo gel(2, 2) irradiated with ultraviolet and Vis lights for 5 min. The gel plate clearly shows back-and-forth motion depending on the wavelength without irradiation history. Moreover, to observe the deformation of the gel with irradiation, we prepare a ribbon-shaped αCD–Azo gel(1, 2). The ribbon-shaped gel turns to a coil by the irradiation of ultraviolet light ( λ =365 nm) from the left side ( Fig. 4g and Supplementary Movie 8 ). The coil-shaped gel returns to the ribbon-shaped gel by Vis light irradiation. The ribbon–coil transition can be repeated at least five cycles. These results indicate that photoisomerization of the Azo group is correlated to the flex behaviour of the αCD–Azo gel plates. The plate or ribbon gels bend in the opposite direction of the incident light because the surface of the gel plate exposed to ultraviolet light expands in water, but the volume of the surface not exposed to ultraviolet light remains constant, suggesting that the strain deformation between the exposed and unexposed areas creates the flex behaviour of αCD–Azo gels. We successfully prepared reversible expansion–contraction supramolecular hydrogels and a supramolecular actuator-like artificial molecular muscle system consisting of αCD–Azo gel. Although microscale switching of supramolecular complexes by external stimuli is well known, achieving a macroscale mechanical change is difficult. Herein, we demonstrate that an intelligent supramolecular actuator could be formed using a main chain with a sufficient length and an adequate number of guest molecules to generate reversible crosslinks between αCD and the Azo units. Although various stimuli and functional groups can be used in responsive materials with host–guest complexes, we chose to employ external photostimuli. Photoisomerization of the Azo group alters the volume of the supramolecular hydrogel by controlling the formation of an inclusion complex. Especially, the plate- and ribbon-like gels showed the shape–memory properties controlled by photoirradiation. Supramolecular hydrogels are important to realize ‘soft machines’ like biological systems. These stimulus-responsive expansion–contraction properties are similar to that of muscle fibrils, such as sarcomere, which consists of actin filaments. Moreover, photoresponsive materials have many general applications, including remotely controlled materials and medical devices. Currently, we aim to achieve a hydrogel system that moves faster and over a larger area. We believe that these stimulus-responsive stretching properties may eventually be used in stents and drug delivery carriers to selectively release drugs. αCD–Azo gels may realize photoresponsive embolization application, where photoresponsive αCD–Azo gels will be introduced into the vessels around a tumour using catheter techniques, and optical fibres will provide the photostimuli. It is hypothesized that the introduced gels will embolize the blood stream in arbitrary vessel positions controlled by photostimuli using optical fibres. Materials α-Cyclodextrin (αCD), βCD and γCD were obtained from Junsei Chemical Co., Ltd. Acetone, methanol, triethylamine, tetrahydrofuran (THF), dimethyl sulfoxide sulphoxide, azobisisobutyronitrile (AIBN), N,N′-methylenebis(acrylamide) and acrylamide were obtained from Nacalai Tesque Inc. Acryloyl chloride was obtained from Wako Pure Chemical Industries, Ltd. A highly porous synthetic resin (DIAION HP-20) used for column chromatography was purchased from Mitsubishi Chemical Co., Ltd. Water used for the preparation of the aqueous solutions (except for NMR measurements) was purified with a Millipore Elix 5 system. Other reagents were used without further purification. Measurements 1 H NMR spectra were recorded at 500 MHz with a JEOL JNM-ECA 500 NMR spectrometer. Chemical shifts were referenced to the solvent values ( δ =2.49 ppm for DMSO and δ =4.79 p.p.m. for HOD). 1 H MAS-NMR spectra were measured at 600 MHz on a VARIAN VNMRJ 600 NMR spectrometer with a sample spinning rate of 1.12~2 kHz and relaxation delay of 10 s at 30 °C. The solid-state 1 H FGMAS (Field Gradient Magic Angle Spinning) NMR spectra were recorded at 400 MHz with a JEOL JNM-ECA 400 NMR spectrometer. Sample spinning rate was 10 kHz. Chemical shifts were referenced to adamantane as an external standard ( δ =1.91 ppm). The infrared spectra were measured using a JASCO FT/IR-410 spectrometer. The ultraviolet–Vis absorption spectra were recorded with a JASCO V-650 and a Hitachi U-4100 spectrometer in water with a 1-mm quartz cell at room temperature. Dynamic viscoelasticity and mechanical properties of the gel were measured using an Anton Paar MCR301 rheometer and mechanical tension testing system (Rheoner, RE-33005, Yamaden Ltd.), respectively. Photoisomerization Azo moieties were isomerized by photoirradiation using a 300 W Xenon lamp (Asahi spectra MAX-301) equipped with suitable mirror modules (ultraviolet mirror module, λ =250–385 nm; Vis mirror module, λ =385–740 nm) as a function of irradiation wavelength. Moreover, to extract specific wavelength, a band-pass filter (LX0365) for ultraviolet light and a band-pass filter (LX0430) for visible light were put on Xenon lamp. The intensities of transmitted ultraviolet light through the band-pass filters (LX0365) using a suitable mirror module is similar for that of Vis light ( λ =430 nm) using the band-pass filter (LX0430). The distance between the sample cell and the lamp was fixed at 10 cm. How to cite this article: Takashima, Y. et al . Expansion–contraction of photoresponsive artificial muscle regulated by host–guest interactions. Nat. Commun. 3:1270 doi: 10.1038/ncomms2280 (2012).